Easy access to medium-sized lactones through metal carbene migratory insertion enabled 1,4-palladium shift Reactions that efficiently construct medium-sized lactones are significant, as they overcome the unfavorable entropic factor and transannular interactions for ring closure, and the lactones produced are common structural motifs recurring in many biologically active compounds. Herein, we describe a valuable strategy for medium-sized lactone synthesis by accomplishing site-selective C–H bond functionalization via a palladium carbene migratory insertion enabled 1,4-palladium shift. The overall process achieves the formal dimerization of two readily available benzaldehyde derivatives, providing value-added products medium-sized lactones. Our method is amenable to late-stage modification of approved drugs and other complex molecules. Mechanistic studies including deuterium-labeling experiments and DFT calculation shed light on the reaction pathways. Palladium/hydride shift [1] , [2] , [3] is an attractive strategy to achieve selective inert C–H bond activation [4] , [5] , [6] , [7] , [8] , [9] , [10] , [11] , [12] , while without the requirement of installing a directing group (Fig. 1a ). This migration event provides a convenient way to activate a specific C–H bond, which might be difficult to achieve by conventional methods. However, for such a fundamental transformation, most studies are focused on migration proceeded within a single molecule [13] , [14] , [15] , [16] , [17] , [18] , [19] , [20] , [21] , [22] , [23] , [24] , [25] , [26] , [27] , which means the reactants involved have to be carefully designed to possess a fitted geometry to undergo the desired migration. Elegant exceptions were reported by Larock and coworkers almost 20 years ago (Fig. 1b ) [28] , [29] , [30] , in which the migration of the palladium moiety took place after an intermolecular reaction of two readily available reactants. The insertion of alkyne was crucial to construct the vinylpalladium intermediate that was ready to undergo corresponding 1,4-palladium migration. Fig. 1: Reaction modes for palladium-catalyzed C–H bond functionalization. a Reaction mode for 1,4-palladium shift. b Alkyne insertion-enabled 1,4-palladium shift. c Proposed metal carbene migratory insertion-enabled 1,4-palladium shift. d Working hypothesis for seven-membered lactone synthesis. Full size image Many feedstock reagents do not contain any directing groups. For related reactions of these compounds, the palladium metal center is too close to the reacting site. The unfavored strain energy makes it is inaccessible to form a palladacycle via direct C–H bond palladation [31] , [32] . Inspired by the seminal work from Larock [28] , [29] , [30] , we propose that whether we can use a modular one-carbon synthon to facilitate the formation of a thermodynamically stable five-membered palladacycle, which in turn realizes the selective C–H bond activation (Fig. 1c ). We believe that the bridging of such a unit to simple reactants may open an avenue for functionalization of inert C–H bonds. In line with our research interests in diazo compounds involved C–H bond activation [33] , [34] , [35] , we assumed that a palladium carbene-enabled acylation [34] for dibenzo-fused seven-membered lactone synthesis could be an ideal probe to test our assumption (Fig. 1d ). In this designed reaction, both reactants could be prepared in multi-gram scale from readily available salicylaldehyde analogs. Studies on palladium carbene participated cross-coupling reactions [36] , [37] , [38] , [39] , [40] support the feasibility of our hypothesis. According to recent discovery, tricylic ring systems possessing a dibenzo structure joined to a central seven-membered lactone show the potential for preventing or treating malignant diseases [41] . Eurotinone, an effective KDR kinase inhibitor, possesses the exact tricylic backbone. Moreover, modular synthesis of these lactones based on traditional methods, such as Baeyer-Villiger (BV) oxidation [42] and macrolactonization [43] , is challenging. As for the BV reaction, the regioselectivity is low when unsymmetric cyclic ketones are employed, and for the latter, multi-step manipulation is required for the synthesis of the particular reactants. As a common feature of intramolecular reactions, the diversity of the products is limited by the ease of synthesis of the reactants. Thus, it is hard to offer large number of samples that are required for massive screening and evaluation by these traditional methods. Here, we report a palladium carbene migratory insertion-enabled medium-sized lactone synthesis [44] . In this reaction, diazo compounds generated in situ are employed as modular dockable building blocks to promote the C–H bond activation. Moreover, this methodology was found to be efficient for late-stage functionalization of complex molecules, which could be useful for fragment-based drug discovery [45] . Reaction development To validate our hypothesis, N -tosylhydrazone 2a was selected as the precursor of bifunctional diazo compound to react with 2-bromobenzaldehyde 1a . 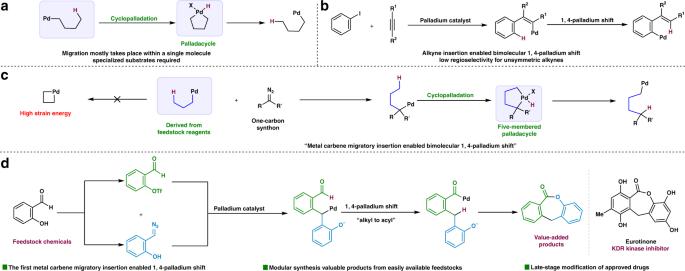Fig. 1: Reaction modes for palladium-catalyzed C–H bond functionalization. aReaction mode for 1,4-palladium shift.bAlkyne insertion-enabled 1,4-palladium shift.cProposed metal carbene migratory insertion-enabled 1,4-palladium shift.dWorking hypothesis for seven-membered lactone synthesis. When the reaction was carried out in THF (tetrahydrofuran) at 80 °C for 10 h, using Pd 2 (dba) 3 •CHCl 3 (2.5 mol%) as palladium source, dppm (bis(diphenylphosphanyl)methane, 7.5 mol%) as ligand, K 3 PO 4 as base, the expected seven-membered lactone 3 was indeed formed in 5% nuclear magnetic resonance (NMR) yield (Table 1 , entry 1). Initial examination of different bidentated phosphine ligands (Table 1 , entries 1–10) found that Xantphos ((9,9-dimethyl-9H-xanthene-4,5-diyl)bis(diphenylphosphane)) performed the best, affording 3 with 80% NMR yield (Table 1 , entry 10). After a brief survey of other palladium sources (Table 1 , entries 11–13) (for a detailed optimization study, see Supplementary Information Table S1 to Table S4 ), we found Pd(OAc) 2 (5 mol%) was ideal. The reaction could complete in a relatively short time, and the corresponding lactone 3 was obtained in 76% isolated yield (Table 1 , entry 11). o -Iodobenzaldehyde 1b could participated in the palladium-catalyzed lactonization as well, the seven-membered lactone 3 was produced in slightly lower NMR yield (entry 14). Table 1 Optimization of reaction conditions for seven-membered lactone synthesis. 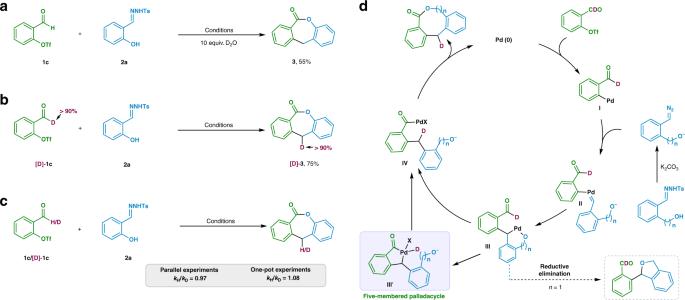Fig. 2: Mechanistic experiments. aReaction proceeded in presence of 10 equiv. of D2O.bDeuterium-labeling experiment as a probe for 1,4-palladium migration.cKinetic isotopic effect experiment for C–H bond cleavage in aldehyde1c.dProposed catalytic cycle for palladium-catalyzed medium-sized lactone synthesis. X stands for possible counter anion. Full size table Substrate scope With the optimized reaction conditions in hand (Table 1 , entry 11), we sought to explore the substrate scope with respect to different o -bromobenzaldehydes and N -tosylhydrazones bearing hydroxy tether (Table 2 ). As depicted, a variety of substituted o -bromoarylaldehydes 1 could participate in current lactonization reaction regardless of the electronic nature of substituents incorporated on the phenyl ring. The corresponding lactones were obtained in moderate to high yields (products 3 – 13 , 65%–84% yields). Sterically hindered 1-bromo-2-naphthaldehyde was also a viable substrate for the reaction, leading to the corresponding product 14 in 55% isolated yield. Table 2 Substrate scope with respect to o -bromoarylaldehydes 1 and N -tosylhydrazones 2 a . Full size table Additional experiments revealed that the current protocol for seven-membered lactone synthesis was efficient, as a wide array of N -tosylhydrazones derived from salicylaldehyde analogs could also react well with 2-bromobenzaldehyde 1a (products 15 – 37 ). Electron-donating (methyl and methoxy, products 15 , 20 , 21 , and 25 ) and electron-withdrawing (chloro, fluoro, even bromo, products 16 – 19 , 22 – 24 , and 26 – 27 ) groups decorated on the aryl ring were tolerated, regardless of the position and steric effects. The tolerance of chloro and bromo groups has offered convenient handle for further transition-metal catalyzed cross-coupling reactions. Functional moieties, such as carbon–carbon triple bond and labile silyl group, stayed intact, and corresponding lactones 28 and 29 were isolated in 67% and 81% yields, respectively. It is worthwhile to mention that N -tosylhydrazone derived from corresponding hydroxylketone was also a viable bifunctional carbene precursor, giving the substituted lactone in moderated yield under a slightly modified condition (product 30 ). The establishment of a chiral carbon center shows the synthetic potential of current method in catalytic asymmetric synthesis, which could be our future research objective. The current lactonization shows potential application on the area of fragment-based drug discovery. As o -hydoxy- N -tosylhydrazones derived from bio-relevant molecules, such as methylparaben, paracetamol, carvacrol, thymol, eugenol, estrone and methyl N -Phth- L -tyrosinate, were competent diazo precursors, and the potentially bioactive ε-lactones 31 – 37 were obtained in moderate to good yields. To further demonstrate the synthetic potential, we proceeded to examine the applicability of our designed chemistry for o -pseudo-halo benzaldehyde substrates instead of 2-bromobenzaldehyde. In principle, both reactants could be availed by exploiting 2-hydroxy benzaldehyde as the same starting material. Treatment of 2-formylphenyl trifluoromethanesulfonate 1c and 2 under the previous optimized conditions (Table 1 , entry 11) produced 3 with 53% of GC yield. Either changing Xantphos to other biphosphine ligands or using other bases instead of K 2 CO 3 did not improve the results. The best result (80% of isolated yield) was obtained when Pd(OAc) 2 was replaced by [Pd(η-C 3 H 6 )Cl] 2 (2.5 mol%) (for a detailed condition experiments, see Supplementary Information Tables S5 to Table S8 ). A feature for current transformation by using o -pseudo-halo aryl aldehydes as the electrophiles is the implementation of formal dimerization of abundant salicylaldehyde analogs to a range of functionalized seven-membered lactones. 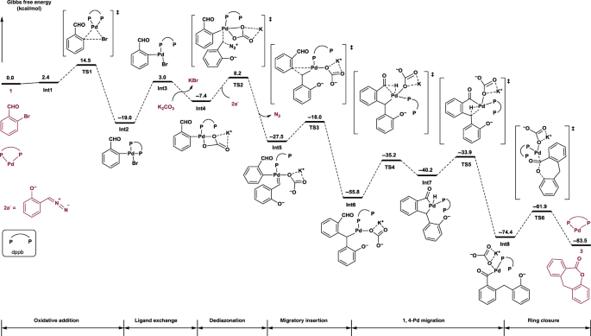Fig. 3: DFT calculations. Reaction energy profiles calculated at M06/def2-TZVP//B3LYP/6-31G(d)(LANL2DZ) level. 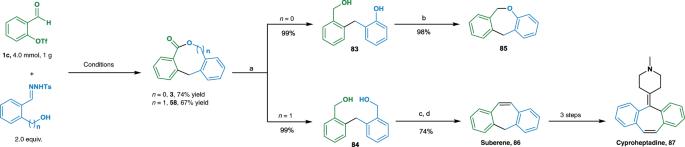Fig. 4: Synthetic manipulations. Reagents and conditions:aLiAlH4, THF, 0 °C, 3 h;bPh3P, diethyl diazene-1,2-dicarboxylate, toluene, 70 °C, 6 h;cDMP,tBuOH, DCM, RT, 5 h;dTiCl4, Zn, pyridine, THF, 0–80 °C, 6 h. Under the optimized conditions we found that both reactants derived from 2-hydroxy benzaldehydes containing a variety of substituents on the phenyl ring could be formally dimerized, giving corresponding lactones in moderate to high yields (Table 3 , products 3 , and 38 – 42 ). Notable examples are those reactants possessing potentially reactive bromo group, could participate in current formal dimerization smoothly (product 41 ). Similarly, the formal cross-dimerization of salicylaldehyde analogs also exhibits very general substrate scope, diverse substituents including electron-donating and electron-withdrawing groups were tolerated, and displayed good orthogonal reactivities of the triflates and N -tosylhydrazones (Table 3 , products 5 , 9 and 43 to 55 ). Alkynyl group and labile trimethylsilyl (TMS) moiety stayed intact under standard reaction conditions (products 56 and 28 ). Table 3 Substrate scope for formal dimerization of salicyaldehyde analogs. a Full size table Current strategy was found applicable for more challenging eight-membered lactone synthesis. Under the optimal conditions for the seven-membered lactone synthesis, we indeed observed the formation of desired lactone 58 ( n = 1) from the reaction mixture, albeit in 15% NMR yield. After identification of the effects of phosphine ligands, palladium sources and bases (for a detailed optimization study, see Supplementary Information Tables S9 – S13 ), the best result with 76% of isolated yield of 58 was obtained with dppb (1,4-bis(diphenylphosphanyl)butane) at 5 mol% Pd loading. It is worthwhile to mention that, for this specific reaction, we have observed the formation of dihydroisobenzofuran as side-product in small amount (5% isolated yield under optimized conditions). This outcome is noteworthy, as the formation of eight-membered lactone 58 , which is generally considered to be energetically less favorable, could override the seemingly favorable pathway for the formation of five-membered compound. This unusual chemo selectivity turned out to be quite general under current conditions for a range of eight-membered lactone synthesis. As the examples shown in Table 3 (products from 57 to 63 ), lactone formation was not significantly affected by the presence of electron-donating or -withdrawing groups on the phenyl ring of the triflates. As exemplified by the products with strongly electron-withdrawing group (product 59 ) and with weakly electron-withdrawing group (product 60 ) were isolated in 70% and 51% yields, respectively. The reactions for the substrates bearing weakly electron-donating group (products 61 and 63 ) and with strongly electron-donating group (product 62 ) proceeded well. Similarly, functional groups, such as TMS and alkynyl groups (product 57 ) were compatible. The abundance of phenolic-derivatives and well-established procedure of ortho -formylation of phenols [46] offered us the opportunity to enrich the substrate scope with lactones having different functionalities. As depicted, the triflates bearing various pharmacophore fragments, such as methylparaben, paracitamol, estrone, eugenol, thymol and methyl N -Phth- L -tyrosinate, could react with salicylaldehyde-derived N -tosylhydrazone under standard conditions, giving the corresponding functionalized bio-relevant seven-membered lactones in 34% to 75% isolated yields (products from 64 to 69 ). For comparison, N -tosylhydrazones derived from methylparaben, eugenol estrone and N -Phth- L -tyrosinate were also tested as the precursors of diazo compounds to react with triflate 1c . Again, the corresponding lactones could be prepared efficiently (Table 3 , products from 31 to 37 , up to 81% isolated yield after column chromatography on silica gel). These potentially bio-relevant reactants were competent substrates for eight-membered homo-analogs synthesis as well. The corresponding lactones containing paracetamol (product 70 ), estrone (products 71 and 72 ), N -Phth- L -tyrosine (product 73 ) and methylparaben (product 74 ) motifs were prepared in moderate to high yields (54–78%). Unambiguous proof of structure and absolute configuration of the bio-relevant lactone 66 was achieved by single-crystal X-ray analysis. Notably, this fragment-based technology was found to be applicable to couple two pharmacophore fragments, giving a variety of complex molecules in a modular fashion (Table 3 , products from 75 – 82 ). The proof-of-concept was firstly expressed by the formal dimerization of estrone and eugenol derivatives under the standard conditions, giving corresponding dimers ( 75 and 79 ) with seven-membered lactone linkers in 74% and 53% isolated yields, respectively. Subsequently, we examined the orthogonal reactivity of both reactants containing pharmacophore structural motifs. Triflate derived from estrone could react with the corresponding N -tosylhydrones prepared from eugenol and methyl N -Phth- L -tyrosinate, and the cross dimerized lactones 76 and 77 were obtained in 43% and 64% isolated yields after chromatography. Following the similar reaction design, highly complex molecules 78 , 80 , 81 , and 82 containing seven-membered lactone scaffolds could be obtained conveniently. Mechanistic investigation In order to gain insights about the reaction mechanism, representative isotopic labeling experiments were carried out. Under otherwise identical conditions, triflate 1c reacted with 2-hydroxy N -tosylhydrazone 2a in presence of 10 equiv. of D 2 O, 3 without any incorporation of deuterium atom was isolated in 55% yield (Fig. 2a ). Whereas, when compound [D]-1c treated with hydrazone 2a under the standard condition, [D]-3 was produced (Fig. 2b ). Finally, the relatively lower value of k H / k D indicated C–H bond cleavage in the aldehyde moiety was not involved in the rate-determining step [47] (Fig. 2c ). Fig. 2: Mechanistic experiments. a Reaction proceeded in presence of 10 equiv. of D 2 O. b Deuterium-labeling experiment as a probe for 1,4-palladium migration. c Kinetic isotopic effect experiment for C–H bond cleavage in aldehyde 1c . d Proposed catalytic cycle for palladium-catalyzed medium-sized lactone synthesis. X stands for possible counter anion. Full size image Taken all the data together, we have proposed a reasonable mechanism for current medium-sized lactone synthesis (Fig. 2d ). The reaction is initiated by oxidative addition of palladium(0) catalyst to o -pseudo-halo benzaldehyde to generate palladium(II) intermediate I . I could be considered as a receptor to react with bifunctional diazo compound, giving palladium-carbene intermediate II . Migratory insertion of II would produce intermediate III , which possesses the exact geometry that is ready to undergo a 1,4-palladium/hydride shift, thus achieving a selective C–H bond activation of the aldehyde moiety [48] . We anticipate such a reaction mode may not be limited to C–H bond activation of an aldehyde moiety. Other functional moieties possessing similar geometry could be applicable for related metal migration. The step for 1,4-palladium migration proceeds in an irreversible manner, since we did not observe any deuterium atom scrambling during the isotopic labeling experiments (Fig. 2b, c ). The fact that no deuterium labeling of 3 occurred when the reaction was carried out in presence of 10 equiv. D 2 O (Fig. 2a ) indicates that H-D exchange between of the potential palladium intermediates and the reaction media is relatively slow. Ring closure of IV generates a high-value medium-sized lactone, where two readily available aldehyde derivatives have been formally dimerized. In the case of eight-membered lactone synthesis, reductive elimination of intermediate III ( n = 1) would give the side-product dihydroisobenzofuran. Density functional theory (DFT) calculations To get more details on the mechanism, a theoretical study of the energy surface of the proposed pathway for the reaction of 1a and 2a catalyzed by a palladium catalyst generated from Pd(OAc) 2 and dppb was carried out by DFT calculations. As shown in Fig. 3 , a weak interaction between Pd complex and reactant 1a is virtually thermoneutral (Δ G = 2.4 kcal/mol). Oxidative addition of 1a to form Int2 is thermodynamically downhill by 21.4 kcal/mol and requires an energy barrier of 12.1 kcal/mol ( TS1 ). To provide a vacant site for further reaction, dissociation of one site of the bidentated ligand is endothermic of 22.0 kcal/mol, yielding Int3 . Ligand exchange of bromide by K 2 CO 3 to form Int4 is an exothermic process. According to our study, the dissociation of dinitrogen is not that facile. Compared to Int2 , the reaction of 2a’ with Int4 has to overcome a barrier of 27.2 kcal/mol ( TS2 ) in energy to generate palladium carbene species Int5 . A subsequent migratory insertion takes place, giving Int6 via a three-membered transition state TS3 , and encountering a low barrier of 9.5 kcal/mol. The C–H activation process starts from Int6 . Palladium atom inserts into the C–H bond of the aldehyde moiety, and produces Int7 , which possesses a five-membered palladacycle with a hydride species sitting on the palladium center. This step presents a barrier of 20.6  kcal/mol ( TS4 ). Hydride transfer from the palladium atom to dibenzylic position has a small barrier of 6.3  kcal/mol. These two steps in whole could be considered as 1,4-palladium/hydride shift, which was consistent with experimental observation of deuterium experiments (Fig. 2b ). For ring closure of Int8 , an outersphere displacement of the palladium moiety by the tethered phenolic anion leads to the formation of final product 3 , which suffers a barrier of 12.5 kcal/mol. Our calculation shows the rate-determining step is dediazonation to form the metal carbene species (from Int2 to Int5 ). Other possible pathways were detailed and discussed in Supplementary Information (See Supplementary Information Fig. S3 ). Fig. 3: DFT calculations. Reaction energy profiles calculated at M06/def2-TZVP//B3LYP/6-31G(d)(LANL2DZ) level. Full size image Synthetic applications The catalytic methods for the synthesis of medium-sized lactones were found to be efficient for large scale of reactions (Fig. 4 ). Thus, when 4 mmol (1 g) of 1c was treated with the bifunctional diazo precursors under optimal conditions, lactones 3 and 58 were obtained in 74% and 67% of isolated yields, respectively. These lactones could be reduced efficiently by LAH, giving the corresponding diols 83 and 84 in quantitative yields. Intramolecular cyclization of 83 would give dibenzo-oxepine 85 . Diol 84 was converted to suberene 86 by using a consecutive DMP oxidation and TiCl 4 -mediated McMurry reaction protocol. To our delight, we found compound 86 has significant utility in preparing miscellaneous medicinally important molecules [49] , [50] , [51] . For example, cyproheptadine 87 , an antihistaminic and antiserotonergic agent, could be prepared by following reported procedures in three steps [52] , [53] . Fig. 4: Synthetic manipulations. Reagents and conditions: a LiAlH 4 , THF, 0 °C, 3 h; b Ph 3 P, diethyl diazene-1,2-dicarboxylate, toluene, 70 °C, 6 h; c DMP, t BuOH, DCM, RT, 5 h; d TiCl 4 , Zn, pyridine, THF, 0–80 °C, 6 h. Full size image In summary, we present a rapid approach to dibenzo-fused seven- and eight-membered lactones. The current palladium-catalyzed medium-sized lactonization is efficient, featuring broad substrate scope, good functional group compatibility, and benefitted by utilization of easily available feedstocks as reactants. From a mechanistic viewpoint, the migratory insertion of palladium carbene is critical, as it afforded the exact palladium(II) intermediate III (Fig. 2d ) possessing a fitted geometry to undergo 1,4-palladium shift. This migration process was further supported by DFT calculations. We believe that such a metal/hydride migration could be a general reaction mode to achieve site-selective C–H bond activation. Further studies following this designed principle are ongoing in our laboratories. General procedure An oven-dried Schlenk tube was cooled to room temperature and filled with argon. To this tube was added Pd(OAc) 2 (5 mol%), Xantphos (7.5 mol%), K 2 CO 3 (3.0 equiv. ), N -tosylhydrazone 2a (0.4 mmol). After the tube was evacuated and refilled with argon three times, 1a (0.2 mmol) and anhydrous THF (2.0 mL) were added. The mixture was stirred at 80 °C. After the reaction was complete (monitored by thin-layer chromatography), the crude mixture was cooled to room temperature, filtered through a short pad of celite and eluented with EtOAc. The resulting solution was concentrated by rotary evaporation. Then, the residual was purified by column chromatography on silica gel to give the pure product 3 .